Pacific deep circulation and ventilation controlled by tidal mixing away from the sea bottom Vertical mixing in the ocean is a key driver of the global ocean thermohaline circulation, one of the most important factors controlling past and future climate change. Prior observational and theoretical studies have focused on intense tidal mixing near the sea bottom (near-field mixing). However, ocean general circulation models that employ a parameterization of near-field mixing significantly underestimate the strength of the Pacific thermohaline circulation. Here we demonstrate that tidally induced mixing away from the sea bottom (far-field mixing) is essential in controlling the Pacific thermohaline circulation. Via the addition of far-field mixing to a widely used tidal parameterization, we successfully simulate the Pacific thermohaline circulation. We also propose that far-field mixing is indispensable for explaining the presence of the world ocean’s oldest water in the eastern North Pacific Ocean. Our findings suggest that far-field mixing controls ventilation of the deep Pacific Ocean, a process important for ocean carbon and biogeochemical cycles. Classical estimates of vertical diffusivity ( Kv ; coefficient of vertical mixing) based on the globally averaged vertical balance of temperature, salinity and chemical tracers in the ocean suggest that 1 × 10 −4 m 2 s −1 of Kv is required to drive the present global thermohaline circulation (THC) [1] . Conversely, measurements around the thermocline (~1,000 m depth) suggest that Kv is typically ~0.1 × 10 −4 m 2 s −1 in many regions and is therefore too small to drive the global THC [2] , [3] . This disparity likely arises because Kv is not uniform but rather highly variable in space; moreover, the heterogeneity of Kv has a significant influence on the global THC [4] , [5] . Since the first evidence for very strong vertical mixing near the rough sea bottom [6] , the relationship between tides and the global THC has been extensively studied [7] , [8] . Tidal flow is forced by periodic changes in the gravitational force in the Earth–Moon–Sun system. Astronomical data suggests that a 3.2 TW loss of rotational energy from the Earth–Moon system (and an additional 0.5 TW loss from the Sun) is converted into tidal energy [9] . Although most of this tidal energy is kinetically dissipated (for example, by bottom friction), it is estimated that around 1 TW of the remaining energy is potentially available for vertical mixing [10] . This means that 1 TW of energy is converted from barotropic (that is, vertically uniform) to baroclinic (that is, vertically nonuniform) tidal flows, which can be used to mix the upper and lower oceans. Previous studies suggest that baroclinic tides generated over the rough sea bottom possess very strong vertical shear, which causes wave breaking and intense vertical mixing there (near-field mixing). Vertical mixing may also be induced away from generation sites; propagating baroclinic tides nonlinearly interact with background internal waves and cascade down to smaller scales, and the resulting vertical shear causes wave breaking (far-field mixing). Such tidal mixing has been considered as a potential driver of the global THC, but questions remain about whether this tidal mixing is sufficient to drive the present-day global THC. A study using numerical simulations with an ocean general circulation model (OGCM) under realistic conditions is essential to quantitatively investigate the above-mentioned question. In previous OGCM simulations, the distribution of Kv induced by tidal mixing was derived from a parameterization such as that proposed by St Laurent et al . [11] However, these OGCM simulations do not necessarily simulate the THC better than the OGCM simulations that employ the classical Kv profile (which is a function of only depth), particularly for the Pacific Ocean [7] , [12] . Furthermore, a recent study suggested that the present tidal parameterization fails to reproduce the observed Kv profiles estimated from microstructure surveys and large-scale hydrographic inversions [13] . Here we shed light on the role of tidal mixing in the global THC by focussing on both mixing near the sea bottom (near-field mixing) and that away from it (far-field mixing). Although previous studies have assumed the latter to merely maintain the background Kv , we propose that this treatment should be modified so that far-field mixing also contributes to the enhancement of Kv with respect to its background value. In this study, we conduct OGCM simulations using the above-mentioned tidal parameterizations and other previously proposed Kv distributions. These results suggest that the Pacific THC can be realistically reproduced by our new parameterization where both near-field and far-field mixing are taken into account. From Δ 14 C simulations, it is clearly demonstrated that our parameterization can capture the observed pattern of the world ocean’s oldest water mass located in the eastern North Pacific Ocean, whereas the previously proposed Kv fails to reproduce its pattern. These results suggest that the far-field mixing is indispensable for controlling the Pacific THC and the ventilation of the deep Pacific Ocean. 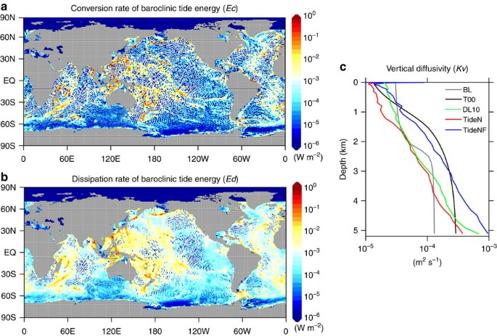Figure 1: Conversion and dissipation rates of baroclinic tide energy and profiles of vertical diffusivity. (a) The depth-integrated energy conversion rate from barotropic to baroclinic tides (Ec). (b) The depth-integrated energy dissipation rate of baroclinic tides (Ed). (c) The globally averaged depth profile of vertical diffusivity (Kv) for BL (gray), T00 (black), DL10 (green), TideN (red) and TideNF (blue). The scale of the lateral axis in (c) is logarithmic. Vertical diffusivity We performed several OGCM simulations listed in Table 1 . Details about model and mixing parameterization are given in the Methods section. In the TideN simulation, in the same way as previous studies, energy conversion rate from barotropic to baroclinic tides ( Fig. 1a ) is used for near-field tidal mixing parameterization. On the other hand, in the TideNF simulation, energy dissipation rate of baroclinic tides ( Fig. 1b ), simulated with a three-dimensional tide model [14] , is also utilized for our new parameterization of far-field tidal mixing. The vertical profile of Kv , applied in TideN (only near-field mixing is included as in previous parameterization) and TideNF (our new parameterization: both near-field and far-field mixing are included) simulations, is displayed in Fig. 1c , which also illustrates several other profiles that are commonly used: a classical one-dimensional profile (BL) [15] , a modified one-dimensional profile (T00) [16] and a roughness diffusion model (DL10) [17] . The T00 profile has larger Kv values below the thermocline than the BL profile. The DL10 profile is obtained from an empirical relationship between Kv and the roughness of the sea bottom, and becomes broadly similar to that of TideN. This similarity was described in a recent comparison study [13] , which pointed out that both the roughness diffusion model and the parameterization of St Laurent et al . [11] appear to underestimate Kv by a factor of ~3 compared with the estimates from hydrographic data inversions. The profile of our TideNF is larger than that of TideN and DL10, but agrees well with the above-mentioned observed estimations. Table 1 Volume transport of THC at the equator. Full size table Figure 1: Conversion and dissipation rates of baroclinic tide energy and profiles of vertical diffusivity. ( a ) The depth-integrated energy conversion rate from barotropic to baroclinic tides ( Ec ). ( b ) The depth-integrated energy dissipation rate of baroclinic tides ( Ed ). ( c ) The globally averaged depth profile of vertical diffusivity ( Kv ) for BL (gray), T00 (black), DL10 (green), TideN (red) and TideNF (blue). The scale of the lateral axis in ( c ) is logarithmic. Full size image Atlantic and Pacific THC The volume transport of the THC reproduced in our OGCM simulations is summarized in Table 1 . Interestingly, differences in the volume transport of the Atlantic THC among simulations are small, and the simulated values are close to the observed estimate [18] in all simulations. This appears consistent with the interpretation proposed by Webb and Suginohara [19] that the strength of the Atlantic THC is controlled by wind stress forcing rather than by the choice of Kv profile. Conversely, the volume transport of the Pacific THC is strongly dependent on the Kv profile selected. The Pacific THC is significantly weaker than the observed estimate in DL10 and TideN, and is also underestimated in BL. Of all the simulations studied, only T00 and TideNF seem to capture the Pacific THC realistically. These results support those obtained in a previous study [16] , which indicates that the value of Kv around the thermocline (~1,000–3,000 m) is key to controlling the strength of the Pacific THC. 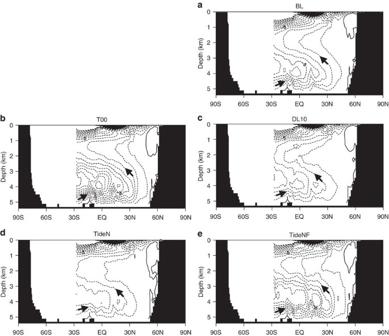Figure 2: Pacific meridional overturning circulation. The meridional overturning stream function in the Pacific Ocean for (a) BL, (b) T00, (c) DL10, (d) TideN and (e) TideNF. Counter interval is 1 Sv (106m3s−1). The black arrows indicate the direction of the ocean circulation. Figure 2 shows the Pacific meridional overturning stream function in each simulation. All simulations capture the basic structure of the Pacific THC: the deep northward inflow of Circumpolar Deep Water from the Southern Ocean, and the mid-depth southward return flow with less upwelling to the surface [18] , [20] . As for the horizontal pattern of the Pacific deep circulation, observations suggest that water separating from the Antarctic Circumpolar Current enters the Pacific Ocean through the Samoan Passage and flows northward along with the bottom western boundary currents [21] . All simulations capture such features of the Pacific deep circulation, although some branches of western boundary currents are not resolved due to coarse resolution. In our simulations, the choice of Kv profile does not significantly change the vertical and horizontal patterns of the Pacific THC, compared with changes observed in the volume transport of the Pacific THC. Therefore, in terms of the Pacific THC volume transport, T00 or TideNF appears most realistic when compared with the observations. Figure 2: Pacific meridional overturning circulation. The meridional overturning stream function in the Pacific Ocean for ( a ) BL, ( b ) T00, ( c ) DL10, ( d ) TideN and ( e ) TideNF. Counter interval is 1 Sv (10 6 m 3 s −1 ). The black arrows indicate the direction of the ocean circulation. Full size image Δ 14 C distributions To evaluate the reproducibility of T00 and TideN more closely, we first compared the simulated temperature and salinity with the observational climatologies [22] . However, differences in their spatial distribution provide very limited information, especially in the deep Pacific Ocean, because temperature and salinity are very uniform in the deep ocean. Therefore, we utilized the distribution of Δ 14 C to assess the reproducibility of the simulations, because Δ 14 C is an excellent indicator of water mass age (that is, how much time sea water spends inside the ocean after sinking from the sea surface). We conducted offline Δ 14 C simulations for individual Kv profiles (see Methods) and compared the simulated distributions with those of the climatology [23] . All simulations captured the inter-basin differences in the climatological Δ 14 C distribution: the water mass is younger in the Atlantic Ocean and older in the Pacific Ocean, and the largest negative values (that is, the oldest water) occur at 2,000–3,000 m in the North Pacific Ocean. This is confirmed in Fig. 3 , which illustrates the climatological and simulated Δ 14 C distribution at 2,500 m depth. However, quantitatively speaking, the magnitude of the largest negative value in the North Pacific Ocean varied between simulations: BL, DL10 and TideN significantly overestimated this value (that is, the water is too old), whereas T00 and TideNF showed better agreement with the climatology. This is consistent with the fact that the strength of the Pacific THC is realistically simulated in T00 and TideNF, whereas the other simulations underestimate it as described above. 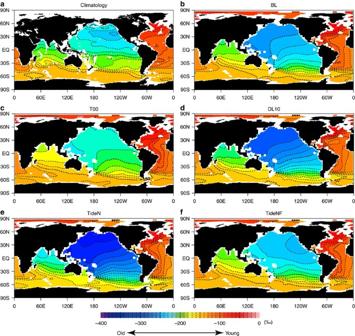Figure 3: Δ14C distribution. (a) The climatological distribution of Δ14C at a depth of 2,500 m. The simulated distribution of Δ14C at a depth of 2,400 m for (b) BL, (c) T00, (d) DL10, (e) TideN and (f) TideNF. The climatology is that of the natural Δ14C provided by Keyet al.23, where the contribution from nuclear explosion has been removed. Figure 3: Δ 14 C distribution. ( a ) The climatological distribution of Δ 14 C at a depth of 2,500 m. The simulated distribution of Δ 14 C at a depth of 2,400 m for ( b ) BL, ( c ) T00, ( d ) DL10, ( e ) TideN and ( f ) TideNF. The climatology is that of the natural Δ 14 C provided by Key et al . [23] , where the contribution from nuclear explosion has been removed. Full size image In the climatology, the oldest water is located around the eastern North Pacific Ocean. TideNF successfully reproduced this pattern, whereas the other simulations (including T00) failed to reproduce it and therein the oldest water was located around the western Pacific Ocean. This indicates that our new parameterization offers significant improvements in the reproducibility of water mass age in the deep Pacific Ocean over the previously proposed Kv profiles. Furthermore, differences between TideN and TideNF clearly demonstrate that tidal mixing by far-field dissipation is essential to control the ventilation of the deep Pacific Ocean. As the ventilation is a key process of the ocean carbon and biogeochemical cycles, our finding implies that far-field mixing also has an important role in such cycles. Parameter sensitivity in tidal mixing parameterization In TideNF, q (efficiency of local dissipation, measure of ratio of near-field to far-field dissipation) and h (vertical decay scale of near-field dissipation) were set to 0.33 and 500 m, respectively. However, their actual values are still unknown, and the values adopted must be chosen from limited observed information [11] . Therefore, we conducted additional OGCM sensitivity simulations (TideNF-series simulations), in which we changed the values of q and h in TideNF systematically ( Fig. 4a,b ). When q was decreased, the volume transport of the Pacific THC increased (green line in Fig. 4a ), suggesting that far-field dissipation can drive the Pacific THC more efficiently than near-field dissipation. The advantages of far-field dissipation driving the Pacific THC result from differences in the vertical structure of dissipation. This was confirmed by comparison with the results for h =100 m (red line in Fig. 4a ) and h =2,000 m (blue line in Fig. 4a ). The volume transport of the Pacific THC significantly changed for h =100 m when we varied q , whereas the Pacific THC became almost independent of q for h =2,000 m. Near-field dissipation cannot efficiently drive the Pacific THC when it is trapped near the sea bottom (that is, when h =100 m), which means that the replacement of far-field dissipation by near-field dissipation (that is, increase of q ) considerably decreases the Pacific THC. Conversely, near-field dissipation can drive the Pacific THC in a similar way to far-field dissipation when it is very loosely trapped near the sea bottom (that is, when h =2,000 m), resulting in almost no dependency of the Pacific THC on the value of q . 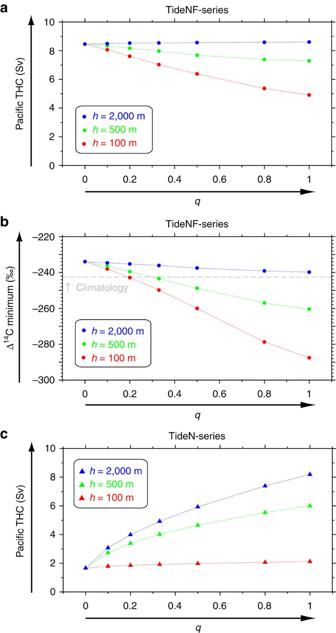Figure 4: Parameter sensitivity in tidal mixing parameterization. (a) The volume transport of the Pacific THC at the equator for TideNF-series. (b) The lowest (oldest) value of Δ14C in the Pacific Ocean for TideNF-series againstq, whereqis efficiency of local dissipation. (c) The volume transport of the Pacific THC at the equator for TideN-series. The red, green and blue symbols representh=100, 500 and 2,000 m, respectively, wherehis vertical decay scale of near-field dissipation. The dashed-grey line in (c) represents the value from the climatology23. Figure 4b summarizes the results of Δ 14 C simulations and suggests that q =0.33/ h =500 m (that is, TideNF) or q =0.2/ h =100 m can simulate the oldest water mass in the Pacific Ocean most realistically. Figure 4: Parameter sensitivity in tidal mixing parameterization. ( a ) The volume transport of the Pacific THC at the equator for TideNF-series. ( b ) The lowest (oldest) value of Δ 14 C in the Pacific Ocean for TideNF-series against q , where q is efficiency of local dissipation. ( c ) The volume transport of the Pacific THC at the equator for TideN-series. The red, green and blue symbols represent h =100, 500 and 2,000 m, respectively, where h is vertical decay scale of near-field dissipation. The dashed-grey line in ( c ) represents the value from the climatology [23] . Full size image To investigate the pure effects of near-field dissipation, we conducted TideN-series simulations in which we systematically varied q and h from the values set in the TideN simulation ( Fig. 4c ). For h =500 and 2,000 m (green and blue lines in Fig. 4c , respectively), the Pacific THC became stronger for larger q , as should be expected from equation 1 (see Methods) where the energy input for tidal mixing is proportional to q . However, for h =100 m, near-field mixing barely contributes to driving the Pacific THC, even for large q (red line in Fig. 4c ). As the value of Kv around the thermocline is important for driving the Pacific THC [16] , near-field dissipation takes place too close to the sea bottom in order to drive the Pacific THC where h =100 m. Conversely, the tidal dissipation can drive the Pacific THC with sufficient efficiency for h =2,000 m, and simulation with q =1 can reproduce the Δ 14 C distribution as well as the TideNF simulation (similar to that shown in Fig. 3f ). However, h =2,000 m is probably inappropriate for near-field dissipation, because a previous study suggested that h =500 m is the upper limit of the vertical scale of near-field dissipation [11] . Furthermore, a recent theoretical study proposed a relationship trade-off: h becomes smaller for more intense near-field dissipation [24] . Although further observational and theoretical studies are necessary, the choice of h =2,000 m could be interpreted as a representative vertical scale for the combination of near-field and far-field dissipation. If this is true, effects of far-field mixing can be easily included into a widely used tidal parameterization merely by setting q =1 with larger vertical decay scale (for example, h =2,000 m). This modification is expected to significantly improve the simulation of the Pacific deep circulation and ventilation. It has been argued that 2 TW of mixing energy is required to drive the global THC and postulated that nearly half of that energy is supplied by tides, with the remaining half supplied by wind-induced internal waves [25] . Such an argument assumes a globally averaged value of Kv , but evidence suggests that the heterogeneity of Kv must be considered for more quantitative discussion. Our results imply that tidal energy alone could drive the global THC; the realistic global THC is reproduced in our TideNF simulation, where 1.1 TW of tidal energy is used to specify the global distribution of Kv . To clarify whether ~1 TW of tidal energy is really sufficient to drive the global THC, more accurate knowledge is required regarding the dissipation processes of tidal energy. In particular, we wish to promote discussion on how much tidal energy is dissipated locally (near-field mixing), how far the remaining tidal energy is propagated away from the generation sites and at which depth the far-field energy is dissipated (far-field mixing). We have demonstrated that far-field mixing can drive the Pacific THC more efficiently than near-field mixing, and suggest that accurate knowledge of the dissipation process of far-field mixing is indispensable for modelling of the global THC. However, the dissipation processes of long-range propagating baroclinic tidal energy that cause far-field mixing remain very unclear both theoretically and observationally. Therefore, in addition to studying the intense mixing near the sea bottom, increased focus should be placed on understanding the dissipation processes of far-field mixing in future studies. In past climates, significant changes in the ventilation of the deep ocean took place: for example, radiocarbon records indicate that the ventilation of the Southern and Pacific Oceans significantly decreased under a glacial climate and could have caused glacial-interglacial changes in atmospheric carbon dioxide concentration [26] . On the other hand, under a future global warming climate, it is anticipated that oxygen-depleted waters, such as those located in the eastern North Pacific Ocean (where the oldest water mass exists), will extend due to the decreased ventilation and exert a serious impact on the ocean's biogeochemical cycles [27] . This study clarifies that the ventilation of the deep Pacific Ocean is controlled by far-field tidal mixing, and therefore, it is implied that tidal mixing will become one of the key factors for discussing the above-mentioned important topics of the ocean's carbon and biogeochemical cycles. We believe that future studies focussing on the role of tidal mixing in the ocean's carbon and biogeochemical cycles will provide us with new insight into past and future climate changes. OGCM simulations The OGCM used is COCO version 4.0 (ref. 28 ). The model has 120 × 128 horizontal grids and 40 vertical layers, and is forced by surface heat, freshwater and momentum flux calculated from a climatological data set for sea surface boundary conditions [29] together with restoration of the sea surface salinity to the climatology [22] . In all simulations, the model is integrated for 4,000 years, and the last 100 years are analysed. The offline Δ 14 C simulations were conducted under monthly averaged ocean circulation and mixing fields obtained from COCO [30] . The distribution of Δ 14 C is determined by advection and mixing in the same way as temperature and salinity, except that internal and surface forcing for Δ 14 C is specified: the value is reduced with a half-life of 5370 years inside the ocean and the surface values are restored to the natural Δ 14 C values provided in the climatology [23] (contribution from nuclear explosion is removed therein). In Δ 14 C simulations, the model is integrated for 5,000 years and the last 100 years is used for the analysis. Tidal mixing parameterization In a widely used tidal mixing parameterization [11] , Kv is expressed as where Kb is background vertical diffusivity, q is local dissipation efficiency, Ec is the rate of energy conversion from barotropic to baroclinic tidal flow, Γ is the mixing efficiency of turbulence, F is a function of the vertical structure of dissipation, ρ is sea water density and N is buoyancy frequency. Variables x, y and z in parenthesis indicate explicitly that Ec and F are horizontally and vertically variable functions, respectively. Here, ρ and N are calculated from temperature and salinity climatologies [22] , and Γ is taken to be 0.2, a widely used value for this parameter [31] . The treatment of the other terms (that is, Kb , q , Ec and F ) is a key part of the parameterization and is described in detail below. To avoid unrealistically large values of Kv , we limit N 2 to be greater than 10 −7 s −2 in weakly stratified regions and density inversions, and prohibit Kv from exceeding 30 × 10 −4 m 2 s −1 in all simulations. In previous studies [7] , [8] , [11] , Ec was empirically derived from the parameterized wave drag term in their barotropic tide model [32] (that is, vertically integrated model). Conversely, in this study, we use Ec explicitly calculated from a three-dimensional tide model [14] ( Fig. 1a ). Despite the differences in the tide model used, the distribution of Ec in the present study is basically the same as that obtained in previous studies [32] . Following St Laurent et al . [11] , F is given as where z is depth ( z>0 ), z b is depth of the sea bottom and h is decay height. In our reference simulation (TideN), we set h to 500 m following St Laurent et al . [11] A recent study suggested that larger values may be more appropriate for mimicking the observed profiles [13] , and it is also suggested that the choice of h has significant effects on the Pacific THC [33] . Therefore, we also conduct sensitivity simulations (TideN-series), where h is set to be smaller (100 m) or larger (2,000 m) than 500 m, in this study. The value of q was commonly set to 1/3rd that in previous studies [7] , [8] , [11] . This means that one third of Ec is dissipated locally and contributes to vertical mixing. The remaining energy (that is, 2/3rds of Ec ) is radiated away from generation sites and is assumed to maintain the background vertical diffusivity ( Kb ). We adopt this approach in our TideN simulation: q and Kb are set to 0.33 and 0.1 × 10 −4 m 2 s −1 , respectively. Although the TideN simulation basically follows the approach defined previously, our TideNF simulation applies the modified parameterization as described below. In TideNF, Kv is parameterized by Here E NEAR is locally dissipated tidal energy (near-field dissipation), which is already included in TideN, while E FAR is remotely dissipated tidal energy (far-field dissipation); F FAR is a function of the vertical structure of far-field dissipation. Although the radiated part of tidal energy (that is, 1− q of Ec ) is assumed to maintain Kb in TideN according to the previous approach, we here assume that this contributes to additional tidal mixing expressed as the third term on the right-hand side of equation 3. Note that we implicitly assume that Kb of 0.1 × 10 −4 m 2 s −1 is maintained by non-tidal energy supplied by wind stress, eddies and so on. In this study, E NEAR and E FAR are expressed as and respectively, where Ed is the vertically integrated dissipation rate of baroclinic tide energy ( Fig. 1b ). Note that the form of Ed diagnosed in the three-dimensional tide model [14] is utilized in our modified parameterization for the first time: Ed has not been able to be diagnosed in previous barotropic tide models. As for the vertical structure, F FAR is not intensified near the sea bottom and is expected to be entirely different to F . Here we simply assume uniform dissipation in the vertical direction: The actual vertical structure of the far-field dissipation depends on wave dissipation processes (for example, wave–wave interaction with the background spectra of internal waves); equation 6 is merely a crude expression of these processes and should be improved in future studies. Tide model The tide model used in this study numerically solves the full three-dimensional Navier–Stokes equations under hydrostatic and Boussinesq approximations [14] . The model is forced by the tidal potential forcing of four major semidiurnal (M2 and S2) and diurnal (K1 and O1) constituents. The model is integrated for 60 days and the last 20 days are analysed. Conversion and dissipation rates of baroclinic tide energy By using results of tidal model simulations, the depth-integrated energy conversion rate from the barotropic to baroclinic tides ( Ec ) is defined as [34] where g is acceleration of gravity, ρ ′ is the deviation of sea water density from the basic field associated with baroclinic tide motions, w s is the vertical velocity resulting from the interaction of barotropic tidal flow with bottom topography, and the overbar denotes the time average. The depth-integrated dissipation rate of baroclinic tide energy ( Ed ) is given by the difference between the energy conversion rate and the energy flux divergence of baroclinic tides [34] : where u′ , v′ and p′ are the eastward and northward velocities and the pressure perturbations associated with baroclinic tidal motions. Note that the global integral of Ed becomes the same as that of Ec , because the energy flux divergence term becomes zero when integrated globally. The globally integrated value of Ec (and Ed ) is very sensitive to the horizontal grid resolution: decreasing the horizontal grid spacing from 1/5° to 1/15°, for example, leads to an increase of the global baroclinic conversion rate from 394 to 782 GW [14] . As this value is expected to be 1,105 GW at the limit of zero grid spacing [14] and comparable to the estimate from satellite altimeter data [10] , Ec and Ed simulated with the finest resolution (1/15°) is multiplied by a factor of 1.5 before being used in this study ( Fig. 1a,b ). In the obtained distribution of Ec ( Fig. 1a ), we can see that the baroclinic tides are effectively generated near coastal regions such over the Indonesian Archipelago, the East China Sea and the Andaman Sea. The energetic baroclinic tides are also generated over the rough sea bottom in the open ocean around the Hawaiian Ridge, the Izu-Ogasawara Ridge, the Polynesia Islands and the Mid-Atlantic Ridges. The distribution of Ed ( Fig. 1b ) is similar to that of Ec but extends more outward from the generation sites of the baroclinic tides as a consequence of wave propagation of baroclinic tidal flows. In the Pacific Ocean, we can see a distinct difference between eastern and western regions: larger dissipation rate is found in the western Pacific Ocean, whereas there is less dissipation in the eastern Pacific Ocean. As discussed in the main text, owing to this east-west difference, TideNF can successfully simulate the realistic ventilation age in the deep Pacific Ocean ( Fig. 3f ). How to cite this article: Oka, A. & Niwa, Y. Pacific deep circulation and ventilation controlled by tidal mixing away from the sea bottom. Nat. Commun. 4:2419 doi: 10.1038/ncomms3419 (2013).